Symmetry breaking in the formation of magnetic vortex states in a permalloy nanodisk The magnetic vortex in nanopatterned elements is currently attracting enormous interest. A priori, one would assume that the formation of magnetic vortex states should exhibit a perfect symmetry, because the magnetic vortex has four degenerate states. Here we show the first direct observation of an asymmetric phenomenon in the formation process of vortex states in a permalloy nanodisk using high-resolution full-field magnetic transmission soft X-ray microscopy. Micromagnetic simulations confirm that the intrinsic Dzyaloshinskii–Moriya interaction, which arises from the spin-orbit coupling due to the lack of inversion symmetry near the disk surface, as well as surface-related extrinsic factors, is decisive for the asymmetric formation of vortex states. Vortices and antivortices are topological excitations with a half-integer skyrmion charge of q=|np /2|=1/2, where n is the winding number and p is the polarity. Vortices have a winding number of n=+ 1 and a polarity of p =±1, whereas antivortices have n =−1 (refs 1 , 2 , 3 ). Magnetic vortices are characterized by an in-plane curling magnetization (chirality) and a nanometer-sized central region with an out-of-plane magnetization (polarity) [4] , [5] , [6] . The latter is defined by a clockwise ( c =1) or counter-clockwise ( c =−1) rotation of the in-plane magnetization. The polarity is the orientation of the core magnetization, either pointing up ( p =1) or down ( p =−1). With two possible orientations of c and p , four different ground states of a magnetic vortex can occur [7] , [8] . The magnetic vortex structure constitutes a fascinating topological structure for fundamental studies of nanoscale spin behaviour and offers great potential as a novel concept in data storage technologies [9] , [10] , [11] , [12] , [13] , [14] , [15] . A priori , one would expect the energy of the four states to be degenerate. A non-degeneracy would not only constitute an unconventional physical phenomenon at the nanoscale but could also lead to potentially interesting applications of magnetic vortices with regard to magnetic sensor or logic elements [16] , [17] . Owing to the lack of experimental techniques enabling simultaneous imaging of in-plane ( c ) and out-of-plane ( p ) magnetic components in nanopatterned structures, most of the experiments on magnetic vortices reported so far have focussed on either the chirality or polarity [9] , [15] . Therefore, the degeneracy of a magnetic vortex has not been experimentally verified to date. Here we report the first experimental result for symmetry breaking in the formation process of vortex states (VSs) in a single circular permalloy (Py, Ni 80 Fe 20 ) nanodisk. The origin of the experimentally observed asymmetric phenomenon is interpreted as the combination of an 'intrinsic' Dzyaloshinskii–Moriya interaction (DMI) arising from the spin-orbit coupling [17] , [18] and surface-related 'extrinsic' factors, such as edge defects, surface roughness, and so on. We utilize full-field magnetic transmission soft X-ray microscopy (MTXM) with high-spatial resolution down to 20 nm (ref. 19 ), because the use of X-ray magnetic circular dichroism for magnetic contrast allow us to observe chirality and polarity simultaneously in a large array of permalloy (Py, Ni 80 Fe 20 ) disks and, therefore, to address the formation process of magnetic VSs in applied external magnetic fields. 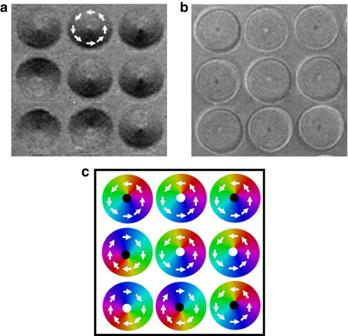Figure 1: Experimental images of vortex structures in Py nanodisk array. MTXM images of in-plane (a) and out-of-plane (b) magnetic components taken at the remanent state in a 100-nm-thick nanodisks. All images were observed in the identical array area. The sense of rotation of the in-plane magnetization is indicated by a white arrow (a). The black and white spots of the central regions in nanodisks are upward and downward vortex cores, respectively (b). The complete vortex configuration of each nanodisk is also illustrated (c). Imaging of magnetic vortex structures Figure 1 shows MTXM images of the in-plane ( Fig. 1a ) and out-of-plane ( Fig. 1b ) magnetic configurations in an identical area of 100-nm thick Py nanodisks with a radius r =500 nm. The dark/bright contrast indicates the projection of the local Fe magnetization along the photon propagation direction of circularly polarized photons. Consequently, the curling in-plane domain structure (chirality), which rotates either clockwise or counter-clockwise, and the small dark or bright spot in the centre of the nanodisks, which represents the upward or downward pointing vortex core (polarity), are clearly visible in Fig. 1a,b . The images were taken at the remanent state (0 mT) after sweeping the external magnetic field from 100 to 0 mT in field steps of 5 mT. The complete vortex configuration of each nanodisk is illustrated in Fig. 1c , where the sequence of the colours indicates the rotation direction of the magnetization in the plane of the nanodisks, and the black and white spots in the centre represent the direction of the vortex core. Obviously, four different VSs, which are defined as c =1 : p =1(S1), c =−1 : p =−1(S2), c =−1: p =1(S3), and c =1: p =−1(S4), are generated in the nanodisks. As the nanodisks are in close proximity to each other with a centre-to-centre distance of d =1,150 nm, one can expect that the dipolar interactions with nearby nanodisks affect the VS formation of each nanodisk within an array. To clarify that assumption, we have studied experimentally the magnetization process of nanodisk arrays with different centre-to-centre distances of d =1200, 1500, 1800 nm. We observed that, with decreasing centre-to-centre distance, the external field for the nucleation of vortices also slightly decreases and the magnetization of nanodisks seems to proceed collectively. One might argue that this results from the dipolar coupling of the nanodisks, but, interestingly, we do not observe the expected correlation in vortex structures of neighbouring nanodisks with regard to the rotation of c and the orientation of p as a function of the centre-to-centre distance. We conclude that dipolar interactions do not have a strong impact on determining the types of VS in individual nanodisks within an array. Figure 1: Experimental images of vortex structures in Py nanodisk array. MTXM images of in-plane ( a ) and out-of-plane ( b ) magnetic components taken at the remanent state in a 100-nm-thick nanodisks. All images were observed in the identical array area. The sense of rotation of the in-plane magnetization is indicated by a white arrow ( a ). The black and white spots of the central regions in nanodisks are upward and downward vortex cores, respectively ( b ). The complete vortex configuration of each nanodisk is also illustrated ( c ). Full size image The complete magnetization-reversal process of Py nanodisks was observed with varying magnetic fields, and a sequence of typical domain structures at magnetic fields from 100, 40, 20, 0, −20, −40, and −100 mT are shown in Fig. 2a . At an external magnetic field of 100 mT pointing in the positive x direction (indicated by the arrow), the nanodisks are fully saturated. By sweeping the applied magnetic field from the saturation field back to 0 mT, magnetic vortices are nucleated, with the vortex cores moving from the edge of the disk towards the centre at 0 mT. With the external field progressing from 0 to −100 mT, the vortex cores shift from the centre to the opposite edges, where they finally annihilate. 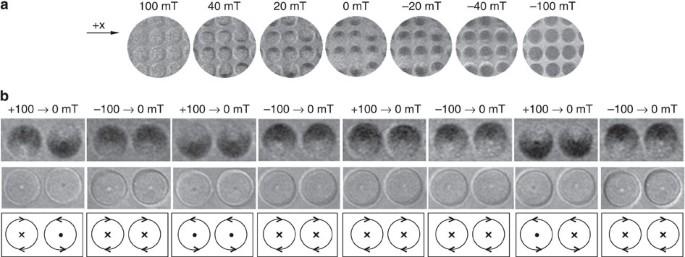Figure 2: Formation process of VSs in repeated measurements. (a) Image sequence of vortex-creation and -annihilation processes driven by an external magnetic field. (b) Chirality and polarity images taken from eight representative images showing two individual nanodisks with a radius of 500 nm and a thickness of 100 nm. The generation rate of each VS group, which is defined as the number of times that each VS group is generated relative to the total number of repetitions, is obviously asymmetric. VSs with a signature ofcp=−1 are predominantly generated compared to VSs withcp=1 with a quantitative generation ratio of 8:0 and 7:1 in the first and second nanodisk, respectively. Figure 2: Formation process of VSs in repeated measurements. ( a ) Image sequence of vortex-creation and -annihilation processes driven by an external magnetic field. ( b ) Chirality and polarity images taken from eight representative images showing two individual nanodisks with a radius of 500 nm and a thickness of 100 nm. The generation rate of each VS group, which is defined as the number of times that each VS group is generated relative to the total number of repetitions, is obviously asymmetric. VSs with a signature of cp =−1 are predominantly generated compared to VSs with cp =1 with a quantitative generation ratio of 8:0 and 7:1 in the first and second nanodisk, respectively. Full size image Symmetry breaking in the formation of vortex states To investigate the symmetric character of the formation process of VSs in individual disks with high statistical significance, we repeatedly recorded MTXM images throughout the process of magnetization reversal in the nanodisk arrays. Figure 2b displays a representative ensemble of eight repeated experiments for c and p in two neighbouring nanodisks, corresponding to 16 independent measurements. Most interestingly, we found that certain types of VSs are dominantly generated, in particular, the formation probability of VS groups with cp =1 (S1, S2: left-handed) and cp =−1 (S3, S4: right-handed) is asymmetric in each nanodisk. To enhance the statistical significance, a total of 50 repeated observations in an array of 30 nanodisks, which yields a total of 1,500 independent measurements, was analysed. Although we found that the dominantly generated VS group for an individual nanodisk can be either cp =1 or cp =−1, we always found an asymmetric generation ratio for the two VS groups. In Table 1 , we list the averaged generation probabilities of VSs, where dominantly (recessively) formed VS groups are denoted as majority (minority). The generation probabilities of majority and minority are found to be 0.71±0.08 and 0.30±0.06, obviously indicating an asymmetry. On the other hand, as also shown in Table 1 , the two VSs belonging to the same VS cp -group are almost symmetrically generated. This result clearly confirms that an experimentally observed symmetry-breaking phenomenon occurs in the formation of two VS groups with different handednesses. This is completely unexpected, assuming that there is equal probability, regardless of handedness, in a single circular nanodisk to generate the four different VSs. Table 1 The averaged experimental generation probabilities of vortex state (VS). Full size table 3D micromagnetic modelling To interpret and explain the asymmetric process of VS formation, we took the DMI into consideration, because it inevitably arises from the spin-orbital coupling due to the broken inversion symmetry at surfaces/interfaces in magnetic thin layers [17] , [18] . The DMI has been discussed as the origin for spin spiral textures and has been theoretically predicted to affect the shape and size of magnetic vortices [20] , [21] . To explore the effect of DMI on the asymmetric formation process of VS, we calculated the generation probabilities of each VS by performing a micromagnetic simulation of the magnetization process of a nanodisk from saturated state to zero-field state. The simulation was carried out with our original code, which was expanded to include the DMI term in the following form: The first and second terms correspond, respectively, to the exchange energy and the magnetostatic energy with the stray field H ms . The last term is DM energy given as where D is the Dzyaloshinskii constant, which determines the magnitude of the DMI and its sign specifies the orientation of spin spiral state owing to the DMI [18] , [20] . For this simulation, we adapted a three-dimensional (3D) model where the DMI exists only on the disk surfaces (top, bottom and lateral) because the DMI is considered to be localized at the surface [18] , [22] , [23] , [24] . A schematic diagram of the 3D modelling is shown in Fig. 3 . The model system is a Py circular disk with r =500 nm and h =100 nm ( Fig. 3a ), which resembles the physical dimensions of the actual disks used in the experiment of Figs 1 and 2 . The mesh size is 4×4×6.25 nm 3 and the DMI is assumed to exist only in the outer meshes, which are shaded in yellow in the side (b) and top view (c) diagrams of Fig. 3 . The coordinates of the DMI components on the lateral and top/bottom surfaces are indicated. In our 3D model, the DMI term on the lateral surface is given in the radial direction, whereas the DMI term on the top/bottom surfaces is given in the z - and angular coordinates in the local cylindrical system. Each coordinate of the DMI on the lateral surface and the DMI on the top/bottom surfaces corresponds to the out-of-plane and in-plane coordinate, respectively. As material parameters for Py, we used M s =8.6×10 5 A m −1 , exchange stiffness A ex =1.3×10 −11 J m −1 , zero magnetocrystalline anisotropy, and damping constant α =1.00. 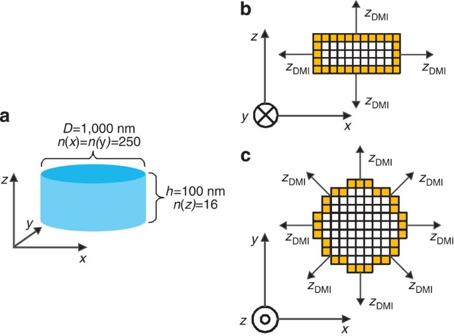Figure 3: Schematic diagram of 3D modelling. (a) The model system is a Permalloy nanodisk with the radius of 500 nm and the thickness of 100 nm divided into a mesh with an element size of 4×4×6.25 nm3. In this model, the DMI is considered to exist only in the outer elements shaded in yellow as shown in side (b) and top (c) view diagrams. The coordinates of the DMI terms on the lateral and top/bottom surfaces given in our 3D model are indicated. Figure 3: Schematic diagram of 3D modelling. ( a ) The model system is a Permalloy nanodisk with the radius of 500 nm and the thickness of 100 nm divided into a mesh with an element size of 4×4×6.25 nm 3 . In this model, the DMI is considered to exist only in the outer elements shaded in yellow as shown in side ( b ) and top ( c ) view diagrams. The coordinates of the DMI terms on the lateral and top/bottom surfaces given in our 3D model are indicated. Full size image Simulation for the generation probability of each VS To investigate the generation probability of each VS under the influence of the DMI, we chose the initial magnetization structure to be a single-domain structure pointing into the same direction (saturated state) by an applied external magnetic field of 150 mT. The external field was decreased from 150 mT with a sweep rate of 1 mT ns −1 until the final state was completed. In the experiment, the change of the magnetization structure was gradual because of the very slow magnetic field sweep rate. On the other hand, a very fast sweep rate had to be used in the simulation because of the limitation of the calculation time. We used a Gilbert damping constant α of 1 to make the change of the magnetization structure gradual with a fast sweep rate, thereby mimicking the experiment. 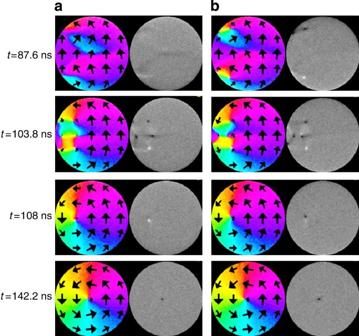Figure 4: Simulated magnetic structures during the magnetization process of a nanodisk. Typical image series of magnetic structures obtained by the simulation for the magnetization process of a nanodisk. In-plane (left) and out-of-plane (right) magnetic structures at each field (time) step are respectively displayed, which are simulated on the top (a) and the bottom layer (b). In the out-of-plane images, the black and white spots represent the down and up polarizations, respectively. Figure 4 illustrates representative image sequences of magnetic structures for the final VS of c =−1: p =−1(S2) simulated at D =1.03×10 −3 J m −2 . The in-plane (left) and out-of-plane (right) magnetization structures observed on the top (a) and bottom (b) layers at each step are displayed, respectively. Interestingly, this simulation provides great detail about the magnetization process of nanodisks, which so far has been completely unexplored. The nucleation of magnetic vortices on the top and bottom surfaces occur asynchronous and unevenly. The cores nucleate from the left side of the bottom layer first ( t =87.6 ns), followed by multiple cores appearing on both layers ( t =103.8 ns). As the magnetization proceeds, a single core with opposite polarity remains on the top and bottom layers ( t =108 ns) and the magnetic structures on both layers become identical. Finally, one of the cores of either the top layer or the bottom layer switches (t =142.2 ns) and the final VS is reached. By varying the DM constant in the simulation, including the case of D =0, we have systematically investigated the nucleation mechanism and magnetization process of VS. At D =0, the generation position of cores are quite random such as left side, right-upper, left-down of disk, and so on. The overall magnetization behaviour of VS sensitively depends on the initial nucleation stage of cores. When the cores appear from one side of disk, the magnetization of VS mostly accompanies with appearing of multiple cores in random positions of disk, while the magnetization proceeds with the moving of created cores when the cores generate on both sides of disk. In the absence of DMI, the same final VS can be defined by different nucleation and magnetization behaviours. At D ≠ 0, the nucleation mechanism is rather simple ( Supplementary Movies 1 ), which might be due to the DMI causing selectivity. The details of the nucleation stage, configuration of multiple cores, motions of cores, annihilating process, and the mechanism of polarity determination can be different, depending on the DM constant. To examine the generation probabilities of each VS, the simulation for the nanodisk magnetization process was repeatedly carried out. We also included thermal noise at T=300 K (ref. 25 ) to introduce stochasticity into our model. The simulation was repeated 200 times for each DM constant and the generation probabilities of cp =1 or −1 were calculated to match the experimental approach. In addition to the simulation with the DMI included on all surfaces, we have also performed the simulation for the case of the DMI existing only on the lateral surface or only on the top and bottom surfaces, respectively. We found that the nucleation mechanism, formation process, and the generation probability of VS are considerably different in each case ( Supplementary Fig. S1 and Supplementary Table S1 ). The results obtained by the simulation with the DMI on all surfaces show comprehensive nucleation and formation processes driven by contributions of all DMI on the lateral surface and top/bottom surfaces. Figure 4: Simulated magnetic structures during the magnetization process of a nanodisk. Typical image series of magnetic structures obtained by the simulation for the magnetization process of a nanodisk. In-plane (left) and out-of-plane (right) magnetic structures at each field (time) step are respectively displayed, which are simulated on the top ( a ) and the bottom layer ( b ). In the out-of-plane images, the black and white spots represent the down and up polarizations, respectively. Full size image The simulation results are summarized in Table 2 . The generation probabilities of the VS groups of cp =1 and cp =−1 are asymmetric and the value of the asymmetry scales with the DM constant. This clearly demonstrates that the DMI has a strong impact on the asymmetric generation of cp =1 or −1. Remarkably, we observe in the simulation that the in-plane magnetization always proceeds in such a way that the chirality with counter-clockwise rotation sense ( c =−1) is generated irrespective of the size of the DM constant and the final state, thereby establishing an unprecedented phenomenon that is due to the DMI. This simulation finding is inconsistent with the experimental result, which observes both chiralities of c =−1 and c =1 ( Figs 1 and 2 ). This difference strongly suggests that surface-related 'external' factors such as edge defects, roughness and geometric variations of individual disks, and so on, might also have an impact on the experimentally observed results in real nanodisks [25] . Thus, the experimental observation that the preferred VS group is different in some nanodisks can be attributed to surface-related external factors to the formation process of VS. Such surface-related defects, which happen to occur inevitably and randomly in individual nanodisks, will affect the magnetization process in particular the nucleation mechanism, which is crucial for the determination of the final state. Therefore, we conclude that both the 'intrinsic' DMI and the surface-related 'extrinsic' factors are important aspects to explain the experimentally observed asymmetric generation behaviour of VS. Table 2 Simulated generation probabilities of vortex states (VS). Full size table To summarize, we have experimentally shown that VSs in a single magnetic nanodisk experience a symmetry breaking in the formation process, which is contrary to the a priori assumption that a magnetic vortex has four different but degenerate ground states. This asymmetric formation process of VS is essential to precisely control the magnetic/spin process in magnetic vortices, which is needed to realize vortex-based data-storage devices. We interpret our experimentally observed asymmetric phenomenon as a consequence of the 'intrinsic' DMI, but we also take surface-related 'extrinsic' factors such as edge defects and/or roughness, ans so on into account. Our results might impact both the fundamental understanding of nanoscale spin behaviour and its potential for technological applications. Sample preparation and MTXM measurement Permalloy (Py) nanodisks with a radius of 500 nm and a thickness of 100 nm were patterned by electron-beam lithography and lift-off process. A total of 30×30 nanodisk arrays with a centre-to-centre distance of d =1,150, 1,200, 1,500 and 1,800 nm were deposited on 100-nm-thick silicon-nitride membranes to allow for sufficient transmission of soft X-rays. Permalloy films were prepared by means of evaporation in an ultrahigh vacuum using an electron-beam gun at a pressure lower than 1×10 −7 Torr. The disks exhibit a polycrystalline structure. Direct observation of vortex structures in Py nanodisks was carried out using full-field MTXM at the Advanced Light Source (beamline 6.1.2.) [19] , enabling real-space magnetic images with high-spatial resolution down to 20 nm. Within an exposure time of a few seconds, a full array of 30×30 disks can be imaged. Magnetic imaging of Py nanodisks was performed at a photon energy corresponding to the Fe L 3 (707 eV) X-ray absorption edge. In MTXM, magnetic contrast is given by X-ray magnetic circular dichroism arising from the dependence of the X-ray absorption coefficients on the orientation between magnetization and photon helicity. To record images of in-plane and out-of-plane magnetizations, specifically the chirality and polarity in the Py nanodisk, the array was mounted at 60 and 90° angles with respect to the X-ray propagation direction, respectively. To reduce non-magnetic background for the in-plane images, images taken at certain fields were normalized to an image recorded in the fully saturated state. The magnetic contrast of the vortex core (out-of-plane configuration) was enhanced by taking images with opposite photon helicities and dividing the two, providing a clear core image with smooth background. How to cite this article: Im, M-Y. et al . Symmetry breaking in the formation of magnetic vortex states in a permalloy nanodisk. Nat. Commun. 3:983 doi: 10.1038/ncomms1978 (2012).